Structural basis of protein phosphatase 2A stable latency The catalytic subunit of protein phosphatase 2A (PP2Ac) is stabilized in a latent form by α4, a regulatory protein essential for cell survival and biogenesis of all PP2A complexes. Here we report the structure of α4 bound to the N-terminal fragment of PP2Ac. This structure suggests that α4 binding to the full-length PP2Ac requires local unfolding near the active site, which perturbs the scaffold subunit binding site at the opposite surface via allosteric relay. These changes stabilize an inactive conformation of PP2Ac and convert oligomeric PP2A complexes to the α4 complex upon perturbation of the active site. The PP2Ac–α4 interface is essential for cell survival and sterically hinders a PP2A ubiquitination site, important for the stability of cellular PP2Ac. Our results show that α4 is a scavenger chaperone that binds to and stabilizes partially folded PP2Ac for stable latency, and reveal a mechanism by which α4 regulates cell survival, and biogenesis and surveillance of PP2A holoenzymes. Protein phosphatase 2A (PP2A) is one of the most important and abundant phospho-Ser/Thr phosphatases in all eukaryotic cells. It forms more than 100 trimeric holoenzymes that target a broad range of cellular substrates, and has a crucial role in many aspects of cellular function [1] , [2] . Each holoenzyme comprises a common core enzyme, formed by a scaffold (A) and a catalytic subunit (C or PP2Ac), and a variable regulatory subunit from four distinct families that controls substrate specificity [1] , [2] . Besides holoenzymes, PP2Ac also associates with a highly conserved regulatory α4 protein that displaces both scaffold and regulatory subunits [3] , [4] , [5] . Mammalian α4 was initially identified as an immunoglobulin-binding protein (IGBP1) [6] and shown to be essential for the survival and maturation of T and B cells [7] , [8] . Conditional knockout of α4 in mouse embryonic fibroblast (MEF) cells showed that α4 is an essential inhibitor of apoptosis [9] . Consistent with this observation, overexpression of α4 has been linked to multiple types of cancer [10] . The yeast homologue of α4, TAP42, is essential for many aspects of cellular function [3] . TAP42/α4 has an important role in the Tor pathway [3] , [11] , [12] and DNA damage response [13] . Interestingly, Tor signalling in turn regulates the level of phosphatase–TAP42 interactions in yeast [3] , [11] . The cellular function of α4 is presumably mediated by its interaction with PP2A and PP2A-like phosphatases, PP4 and PP6 ( [14] ), which share a high degree of sequence similarity ( Supplementary Fig. S1 ) and regulatory mechanisms with PP2A. Despite intense study, the mechanism of α4 in phosphatase regulation remained elusive. Mammalian α4 was initially suggested to be a regulatory subunit that inhibits PP2A activity towards some substrates, but augments its activity towards others [15] , [16] , [17] . More recently, α4 was shown to protect PP2A from poly-ubiquitination and degradation [13] , [18] . Although α4 binds exclusively to PP2Ac and the α4-bound phosphatase is inactive, it was shown to be essential for the formation, stability, and activity of all PP2A complexes [13] , underlying the function of α4 in stable PP2A latency. Understanding the mechanism of α4 function relies on the high-resolution structure of α4 bound to PP2Ac, which, however, had been very slow to emerge. Here we report the structural basis of α4 interaction with PP2Ac and link their contacts to the cellular function of α4. Intriguingly, the α4-binding site is absent in active PP2Ac, but can be induced by dislodging catalytic metal ions or constitutively exposed in an N-terminal fragment of PP2Ac (nPP2Ac, 1–153). The crystal structure of nPP2Ac bound to α4 shows that α4 binding involves PP2A internal packing near the phosphatase active site, which requires local unfolding of a ‘helix switch’ and ‘loop switch’. This stabilizes an inactive conformation of the active site and leads to an allosteric relay through the central β-sheet that alters the scaffold subunit-binding site at the opposite surface. Our study demonstrates that α4 binds selectively to and stabilizes the partially folded PP2Ac for stable PP2A latency, which underlies an important molecular basis for the role of α4 in cell survival and phosphatase regulation. Crystallization of nPP2Ac bound to α4 Initial efforts to determine the crystal structure of the PP2Ac–α4 complex were hampered by the lack of interaction between α4 and the purified recombinant active PP2Ac in vitro ( Supplementary Fig. S2a,b ). Based on reports that the interaction between PP2Ac and α4 was increased by heat shock [5] , [13] and our recent data that suggested a malleable nature of PP2Ac following eviction of catalytic metal ions [19] , we tested the possibility that α4 binds selectively to the partially folded PP2Ac. Co-incubation with pyrophosphate (PPi) at 37 °C rapidly dislodges PP2A catalytic metal ions as indicated by ICP-MS (inductively coupled plasma mass spectrometry), resulting in rapid formation of a stoichiometric complex between PP2Ac and α4 accompanied by a nearly complete loss of phosphatase activity ( Fig. 1a ). α4 binding in turn prevented rapid aggregation of PP2Ac upon dislodging of catalytic metal ions ( Fig. 1b ). These results are consistent with our notion that PP2Ac is partially folded in the absence of catalytic metal ions, which allows α4 binding that in turn prevents aggregation, presumably by shielding exposed PP2Ac internal packing. The resulting PP2Ac–α4 complex, however, eluded crystallization despite considerable effort. 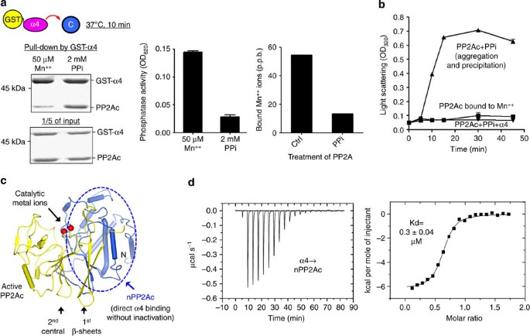Figure 1: Selective binding of α4 to the partially folded PP2Ac. (a) Pull-down of PP2Ac by GST-α4 after co-incubation at 37 °C in the presence of 50 μM Mn++or 2 mM PPi (left panel), the level of the phosphatase activity measured at the end of incubation (middle panel) and changes in the level of Mn++ions stably bound to PP2Ac before and after PPi treatment (right panel). Experiments were repeated three times; representative results are shown. Phosphatase assay was performed in triplicates and mean±s.e.m. were calculated and shown. (b) Light scattering detected aggregation of PP2Ac upon PPi treatment (PP2Ac+PPi), which is suppressed by the presence of α4 (PP2Ac+PPi+α4). (c) Illustration of nPP2Ac using the structure of active PP2Ac. (d) Determination of the binding affinity between nPP2Ac and α4 using ITC. Figure 1: Selective binding of α4 to the partially folded PP2Ac. ( a ) Pull-down of PP2Ac by GST-α4 after co-incubation at 37 °C in the presence of 50 μM Mn ++ or 2 mM PPi (left panel), the level of the phosphatase activity measured at the end of incubation (middle panel) and changes in the level of Mn ++ ions stably bound to PP2Ac before and after PPi treatment (right panel). Experiments were repeated three times; representative results are shown. Phosphatase assay was performed in triplicates and mean±s.e.m. were calculated and shown. ( b ) Light scattering detected aggregation of PP2Ac upon PPi treatment (PP2Ac+PPi), which is suppressed by the presence of α4 (PP2Ac+PPi+α4). ( c ) Illustration of nPP2Ac using the structure of active PP2Ac. ( d ) Determination of the binding affinity between nPP2Ac and α4 using ITC. Full size image We then turned our efforts to identify a sub-domain of PP2Ac that constitutively exposes the α4-binding site. Extensive test based on the structure of active PP2Ac (PDB accession code: 2IE3 ) led to identification of an N-terminal fragment of PP2Ac (nPP2Ac, residues 1–153) that was successfully expressed in a soluble form and bound to α4 without incubation at 37 °C. This partial PP2Ac encompasses the compact N-terminal helix motif and the closely packed β-strands in the first layer of the two central β-sheets ( Fig. 1c ). The binding affinity between nPP2Ac and α4 was 0.3 μM measured by isothermal titration calorimetry (ITC) ( Fig. 1d ). In contrast, ITC barely detected any interaction between active PP2Ac and α4 ( Supplementary Fig. S2b ). Thus, nPP2Ac resembles the partially folded PP2Ac in exposing the α4-binding site. This interaction is highly conserved, as TAP42 could replace α4 for interaction with nPP2Ac ( Supplementary Fig. S2c ). After extensive efforts, an nPP2Ac–α4 complex was crystallized and the structure was determined by Se-Met SAD (single-wavelength anomalous dispersion), and refined to 2.8 Å ( Supplementary Table 1 ). Although we had attempted molecular replacement using the structure of TAP42 or α4 (PDB accession codes: 3QC1 and 2V0P ) [20] , [21] , and a partial structure derived from active PP2Ac (PDB accession code: 2IE3 ) [22] , no solution was obtained, likely due to large conformational changes in the nPP2Ac–α4 complex. Overall structure of the nPP2Ac–α4 complex The structure of the nPP2Ac–α4 complex showed that a pair of widely opened helix tweezers formed by helix 5 and 6 in α4, 45 Å and 55 Å in length, respectively, clamp onto the ends of the helix motif of nPP2Ac ( Fig. 2a ). The α4 helix tweezers are more open in the α4 apo-structure [21] , but adopt a relatively closed conformation by interaction with nPP2Ac. Little change is observed for the PP2Ac helix motif compared with active PP2Ac, suggesting that folding of this helix motif remains intact in the partially folded PP2Ac. One of the helices (C63–69) is relaxed into an extended strand, likely induced by crystal packing ( Fig. 2a ). 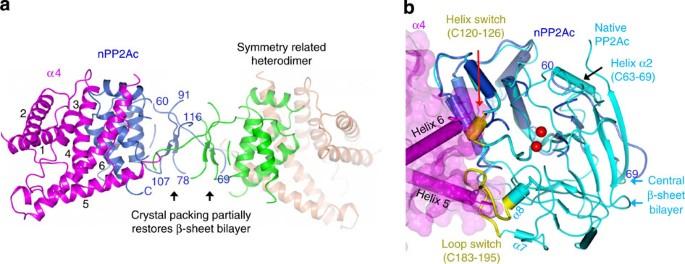Figure 2: Overall structure of the nPP2Ac–α4 complex. (a) Overall structure of the nPP2Ac–α4 complex and the symmetry-related heterodimer in ribbon. The nPP2Ac, α4 and their symmetry-related counterparts are coloured blue, magenta, green, and orange, respectively. (b) Structural overlay of the nPP2Ac–α4 complex and the active PP2A catalytic subunit (PDB accession code:2IE3) by the N-terminal helix motif. The colour scheme is the same as ina, except that active PP2Ac is coloured cyan and the helix and loop switches are coloured yellow. Helices and β-strands are shown in tube and ribbon, respectively. α4 is shown in semi-transparent surface. Only helix 5 and 6 of α4 are shown in tube. Red spheres represent catalytic metal ions in active PP2Ac. Figure 2: Overall structure of the nPP2Ac–α4 complex. ( a ) Overall structure of the nPP2Ac–α4 complex and the symmetry-related heterodimer in ribbon. The nPP2Ac, α4 and their symmetry-related counterparts are coloured blue, magenta, green, and orange, respectively. ( b ) Structural overlay of the nPP2Ac–α4 complex and the active PP2A catalytic subunit (PDB accession code: 2IE3 ) by the N-terminal helix motif. The colour scheme is the same as in a , except that active PP2Ac is coloured cyan and the helix and loop switches are coloured yellow. Helices and β-strands are shown in tube and ribbon, respectively. α4 is shown in semi-transparent surface. Only helix 5 and 6 of α4 are shown in tube. Red spheres represent catalytic metal ions in active PP2Ac. Full size image The single layer β-sheet in nPP2Ac self-associates at the crystal packing interface and partially restores the bilayer architecture in full-length PP2Ac ( Fig. 2a , Supplementary Fig. S3 ). Unlike the helix motif, the β-strands in nPP2Ac are shifted, and the three active site loops and metal-chelating residues within these loops are largely disordered and invisible ( Fig. 2a ). These changes might reflect those in the partially folded PP2Ac. As binding of catalytic metal ions is required to stabilize the active site loops and enzyme structure, it is conceivable that the absence of catalytic metal ions might affect the conformation of the active loops and the central β-sheets that are directly linked to these loops. The structure of the nPP2Ac–α4 complex provides an important opportunity to elucidate changes in PP2Ac required for α4 binding. Alignment of active PP2Ac (PDB accession code: 2IE3 ) and the nPP2Ac–α4 complex via the unaltered helices revealed that two structural elements in active PP2Ac near the phosphatase active site need to be unfolded to allow α4 binding: a small helix (C120–126, helix switch) and an extended loop (C183–195, loop switch) ( Fig. 2b ). Dynamics of helix and loop switch in the α4-bound PP2Ac To corroborate the structural observation, we examined the dynamic nature of the helix and loop switch in the α4-bound PP2Ac using hydrogen–deuterium (H–D) exchange mass spectrometry (MS). For active PP2Ac (stabilized by Mn ++ ), the peptides encompassing the helix switch and its neighbouring active site loop (86–95) exhibited the highest level of backbone amide deuterium intake among all the detected PP2Ac peptides ( Fig. 3a ), indicating that the helix switch is already dynamic in active PP2Ac. The level of deuterium intake into the α4-bound PP2Ac was compared with active PP2Ac ( Fig. 3b ). Two buried peptides in active PP2Ac encompassing central β-strands (residues150–158 and 256–265) exhibit the highest increase in deuterium intake upon binding to α4, indicating that PP2Ac central structures become dynamic in the α4-bound PP2Ac. One of these peptides (residues150–158) is buried by the loop switch in active PP2Ac, consistent with the structural observation that α4 binding requires local unfolding of the loop switch ( Fig. 2b ). Collectively, the results of H–D exchange support our notion that the structure of nPP2Ac–α4 complex reflects the interaction between PP2Ac and α4. 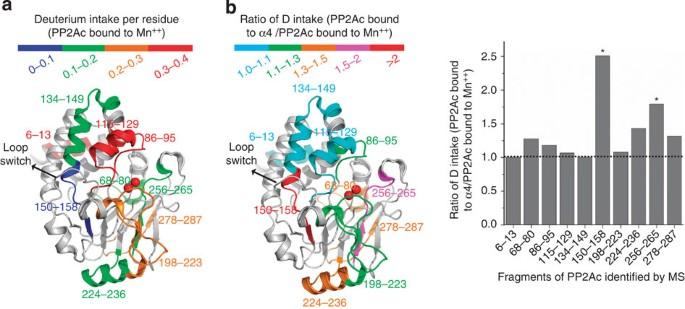Figure 3: H–D exchange analysis of PP2Ac. (a) The structure of PP2Ac with colour code indicating the level of backbone amide deuterium intake into active PP2Ac peptides. (b) Ratio of backbone amide deuterium intake of PP2Ac bound to α4 versus active PP2Ac (bound to Mn++). Stars indicate the two peptides with highest increase in backbone amide deuterium intake when bound to α4. Colour-coded results are illustrated on the structure of PP2Ac (left). Figure 3: H–D exchange analysis of PP2Ac. ( a ) The structure of PP2Ac with colour code indicating the level of backbone amide deuterium intake into active PP2Ac peptides. ( b ) Ratio of backbone amide deuterium intake of PP2Ac bound to α4 versus active PP2Ac (bound to Mn ++ ). Stars indicate the two peptides with highest increase in backbone amide deuterium intake when bound to α4. Colour-coded results are illustrated on the structure of PP2Ac (left). Full size image Displacement of PP2Ac internal packing The helix and loop switch directly contact each other and fold against the N-terminal helix motif in active PP2Ac (PDB accession code: 2IE3 ) [22] ( Fig. 4a ). The underlying internal packing required for α4 binding is clustered at two arginine centres ( Fig. 4b ). At the first arginine centre of active PP2Ac, Arg185 in loop switch makes extensive intramolecular H-bond interactions to the backbone carbonyl groups of residues 40, 42 and 152 and the sidechain of Asn44, buttressed by hydrophobic contacts made by Leu186 in loop switch to Thr40 and Tyr152. In the nPP2Ac–α4 complex, Arg155 of α4 occupies the same position as Arg185 in PP2A loop switch, making similar intermolecular contacts, and Ile159 of α4 replaces internal hydrophobic contacts of Leu186 in PP2A loop switch and forms intermolecular contacts to the same PP2Ac residues ( Fig. 4b ). At the second arginine centre of active PP2Ac, Arg121 in helix switch makes extensive intramolecular H-bond and salt-bridge interactions to three acidic residues, Asp148, Asp151, and Glu188, buttressed by an H-bond formed by Thr122 and Trp143 ( Fig. 4b ). Arg121 also interacts with Glu188, contributing to internal packing between helix (Arg121) and loop switch (Glu188) ( Fig. 4b ). Relaxation of helix switch disrupts the internal packing of Arg121 and allows similar intermolecular H-bond and salt-bridge network to be formed between Lys158 of α4 and Asp148/151 of PP2Ac ( Fig. 4c ). It also allows van der Waals contacts between Trp143 of PP2Ac and at least four residues in α4 ( Fig. 4c ). 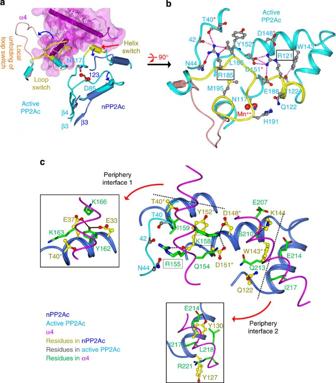Figure 4: Characterization of the PP2Ac–α4 interface and displacement of PP2A internal packing. (a) Illustration of the displacement of the loop switch and helix switch between active PP2Ac and the α4 complex. Structural presentations and the colour scheme are the same as inFig. 2b, except that the loop switch in the partially folded PP2Ac is coloured coral. (b) A close-up view of PP2A internal packing displaced by α4 binding clustered at two arginine centres. Structure presentations and the colour scheme are the same as ina, except that active PP2Ac is shown in ribbon. Residues from active PP2Ac are in ball-and-stick and coloured grey. (c) A close-up view of the PP2Ac–α4 interface involving regions of PP2A internal packing and direct contacts with PP2A surface residues at two periphery interfaces (inlets). The structural orientation is the same as inb. The nPP2Ac and α4 are in ribbon and worm, respectively. Residues of α4 and nPP2Ac are in ball-and-stick and cylinder and coloured green and yellow, respectively. Figure 4: Characterization of the PP2Ac–α4 interface and displacement of PP2A internal packing. ( a ) Illustration of the displacement of the loop switch and helix switch between active PP2Ac and the α4 complex. Structural presentations and the colour scheme are the same as in Fig. 2b , except that the loop switch in the partially folded PP2Ac is coloured coral. ( b ) A close-up view of PP2A internal packing displaced by α4 binding clustered at two arginine centres. Structure presentations and the colour scheme are the same as in a , except that active PP2Ac is shown in ribbon. Residues from active PP2Ac are in ball-and-stick and coloured grey. ( c ) A close-up view of the PP2Ac–α4 interface involving regions of PP2A internal packing and direct contacts with PP2A surface residues at two periphery interfaces (inlets). The structural orientation is the same as in b . The nPP2Ac and α4 are in ribbon and worm, respectively. Residues of α4 and nPP2Ac are in ball-and-stick and cylinder and coloured green and yellow, respectively. Full size image The contacts with PP2Ac internal packing constitute the bulk central region of the nPP2Ac–α4 interface, which is buttressed by α4 contacts with the fully exposed PP2Ac surface residues at two peripheral arms ( Fig. 4c ). At one arm, Glu33 and Glu37 in PP2Ac make several H-bond interactions with Tyr162 of α4. At the other arm, Tyr130 in PP2Ac makes hydrophobic contacts with Ile217 and Leu218 in α4 and H-bond interaction with α4 acidic residues, Glu214. The later in turn makes a salt-bridge interaction with Lys144 of PP2Ac. Collectively, the nPP2Ac–α4 interface buries 1800 Å 2 of surface area, half of which involves PP2Ac internal packing. The nPP2Ac–α4 interface explains previous observations on phosphatase-α4 interactions. A majority of PP2Ac residues at the interface with α4 are the same as those in PP4c and PP6c ( Supplementary Fig. S1 ), consistent with previous observations that α4 specifically regulates the function of all PP2A-like phosphatases [13] , [14] , [20] . Double mutation of TAP42 (R163E/K166D) or human α4 (R155E/K158D) abolished its interaction with PP2A and PP6 and compromised the function of α4 in protecting PP2A from degradation [18] , [20] . Both of these residues contact PP2Ac internal packing at the nPP2Ac–α4 interface ( Fig. 4b ). Arg155 and Lys158 are located in helix 5 of α4 that adopts various conformations in TAP42 dramatically different from α4 apo-structure [20] , [21] . Despite these structural variations, TAP42 and α4 bind to nPP2Ac equally well ( Supplementary Fig. S2c ). Structural alignment shows that helix 5 in the open form of TAP42 (MolA) overlaps with helix 5 of the nPP2Ac-bound α4 ( Supplementary Fig. S4a ). This supports TAP42 interaction with nPP2Ac, but neither forms of TAP42 would interact with active PP2Ac. Helix 5 in α4 apo-structure has minor clashes with active PP2Ac, but is placed near a patch of basic and hydrophobic surface of active PP2Ac ( Supplementary Fig. S4b ). The underlying repulsive contacts explain why α4 could not bind directly to active PP2Ac despite its ability to adopt a widely opened conformation. α4 stabilizes an inactive conformation of the active site One important consequence of displacement of PP2A helix and loop switch and α4 binding is that the PP2Ac active site is stabilized in an inactive conformation. The helix switch is connected to the PP2Ac active site loop harbouring metal-chelating residue Asn117, and juxtaposed to another active site loop that harbours metal-chelating residue Asp85 in active PP2Ac. Both loops are intrinsically dynamic as indicated by H–D exchange ( Fig. 3a ). In the nPP2Ac–α4 complex, both active site loops and metal-chelating residues are largely disordered and restricted in a distorted conformation ( Fig. 4a ). To determine whether the α4-bound PP2Ac is indeed stabilized in an inactive conformation, we purified the α4-bound full-length PP2Ac generated by PPi treatment over gel filtration column to remove PPi and free metal ions, followed by measurement of the phosphatase activity with and without re-activation by Mn ++ ( Supplementary Fig. S5a ). Addition of Mn ++ barely restored the phosphatase activity of the inactive complex that could barely associate with Mn ++ ions ( Supplementary Fig. S5b ). This result is consistent with the structural observation that the α4-bound PP2Ac is stabilized in an inactive conformation that cannot bind metal ions. Exclusive binding of α4 and PP2A scaffold subunit Previous studies suggested that α4 and the scaffold subunit bind mutually exclusively to PP2Ac ( [5] ). Strikingly, structures of the nPP2Ac–α4 complex and PP2A core enzyme [22] show that α4 and the scaffold subunit bind to opposite sides of PP2Ac and do not overlap ( Fig. 5a ). We hypothesize that exclusive binding of α4 and the scaffold subunit is mediated by allosteric changes through PP2A inner structures ( Fig. 5a ). The first central β-sheet of PP2Ac connects to the active site loops and the helix switch at one end, and to the scaffold-binding site at the other end [22] . Unfolding of helix switch and perturbation of active site loops would lead to shift of the central β-sheet that in turn alters the scaffold subunit-binding site at the opposite end. These changes favour α4 binding but weaken scaffold subunit binding. 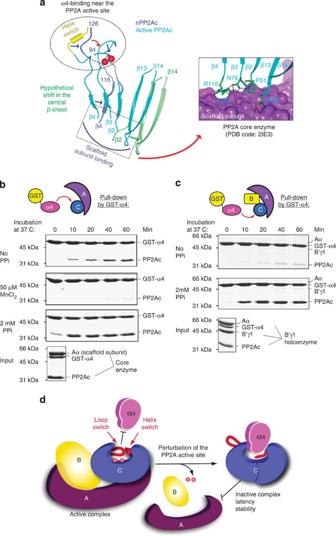Figure 5: Exclusive binding of α4 and the scaffold subunit. (a) Illustration of allosteric relay from the α4-binding site, the helix switch, the active site loops and the first central β-sheet, to the scaffold subunit-binding sites at the opposite end of the β-sheet. Hypothetical shift of the central β-sheet is shown in green. A portion of the interface between PP2A scaffold and catalytic subunits is shown (right). Structural presentations and colour scheme are similar toFig. 4a. The scaffold subunit is shown in surface and coloured purple. Residues of the catalytic subunit are in cylinder and coloured green. (b) Time-dependent conversion of PP2A core enzyme to the α4-PP2Ac complex in the presence and absence of 50 μM Mn++or 2 mM PPi, determined by pull-down via GST-α4. The bound protein samples were visualized on SDS–PAGE by Coomassie blue staining. (c) Time-dependent conversion of stable B′γ1 holoenzyme to the α4-PP2Ac complex in the presence and absence of 2 mM PPi. Experiments were performed similar tob. For panelsbandc, experiments were repeated three times; representative results are shown. (d) Schematic diagram of the structural basis for conversion of active PP2A oligomeric complexes to inactive α4 complex. Disturbance of the active site and dislodging of catalytic metal ions (red spheres) lead to relaxation of the helix switch and loop switch, which allows α4 binding and alters the scaffold subunit-binding site at the opposite surface through allosteric changes propagated through central structures. A, B and C stand for PP2A scaffold, regulatory, and catalytic subunits, respectively. Figure 5: Exclusive binding of α4 and the scaffold subunit. ( a ) Illustration of allosteric relay from the α4-binding site, the helix switch, the active site loops and the first central β-sheet, to the scaffold subunit-binding sites at the opposite end of the β-sheet. Hypothetical shift of the central β-sheet is shown in green. A portion of the interface between PP2A scaffold and catalytic subunits is shown (right). Structural presentations and colour scheme are similar to Fig. 4a . The scaffold subunit is shown in surface and coloured purple. Residues of the catalytic subunit are in cylinder and coloured green. ( b ) Time-dependent conversion of PP2A core enzyme to the α4-PP2Ac complex in the presence and absence of 50 μM Mn ++ or 2 mM PPi, determined by pull-down via GST-α4. The bound protein samples were visualized on SDS–PAGE by Coomassie blue staining. ( c ) Time-dependent conversion of stable B′γ1 holoenzyme to the α4-PP2Ac complex in the presence and absence of 2 mM PPi. Experiments were performed similar to b . For panels b and c , experiments were repeated three times; representative results are shown. ( d ) Schematic diagram of the structural basis for conversion of active PP2A oligomeric complexes to inactive α4 complex. Disturbance of the active site and dislodging of catalytic metal ions (red spheres) lead to relaxation of the helix switch and loop switch, which allows α4 binding and alters the scaffold subunit-binding site at the opposite surface through allosteric changes propagated through central structures. A, B and C stand for PP2A scaffold, regulatory, and catalytic subunits, respectively. Full size image Consistent with this notion, perturbation of the PP2A active site by incubation with 2 mM PPi leads to rapid switch of the PP2A core enzyme (AC complex) to the GST-tagged α4/PP2Ac complex at 37 °C ( Fig. 5b ). The presence of 50 μM Mn ++ ions, which helps to stabilize the active site, inhibited slow conversion of PP2A core enzyme to the GST-α4/PP2Ac complex. No scaffold subunit was associated with the PP2Ac–α4 complex, supporting exclusive binding of α4 and the scaffold subunit. A weakened interaction between the scaffold and catalytic subunits is expected to also destabilize the trimeric holoenzyme. Co-incubation of GST-α4 and the holoenzyme containing B′γ1 at 37 °C in the presence of 2 mM PPi led to rapid conversion of the holoenzyme to the GST-α4/PP2Ac complex, excluding both the scaffold and B′γ1 regulatory subunits ( Fig. 5c ). Conversion of the holoenzyme could be barely observed in the absence of PPi. The much lower rate of holoenzyme conversion compared with the core enzyme reflects the higher stability of the holoenzyme. This suggests that PP2Ac that cannot form stable holoenzymes would have a greater tendency to associate with α4. This explains why mutation of PP2Ac that disrupted binding of the scaffold subunit led to an increased association with α4 ( [5] ). α4-phosphatase interface dictates the role of α4 in survival To determine if the PP2Ac–α4 interface predicted from the structure of nPP2Ac–α4 complex is essential for α4 function, we identified α4 mutations that disrupted PP2Ac interaction. As shown by pull-down assay ( Fig. 6a ), α4 mutations, R155E and K158D at the interface with PP2Ac internal packing and Y162D and E214R at the interface with PP2Ac surface residues, completely abolished the interaction between α4 and the GST-tagged nPP2Ac. In contrast, a mutation located outside the nPP2Ac–α4 interface, E206R, barely affected the interaction. Consistent with the in vitro binding results, recombinant Flag-tagged α4 harbouring mutations at either interface, R155E and E214R, had severely reduced interaction with the cellular full-length PP2Ac ( Fig. 6b ). 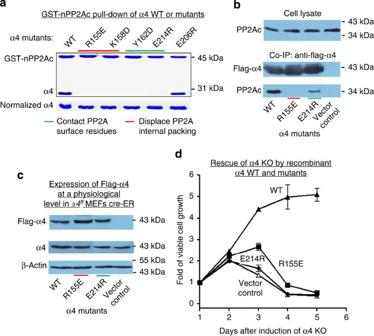Figure 6: The α4 interfaces with the phosphatase are essential for the role of α4 in cell survival. (a) Mutational analysis of α4 residues at the interface with both PP2A internal packing and surface residues. Pull-down assay determined the effect of α4 mutations on interaction between α4 and GST-nPP2Ac. Proteins bound to GS4B resin were visualized on SDS–PAGE by coomassie blue staining. (b) Co-IP showed defects of recombinant Flag-α4 mutants in binding to cellular PP2Ac in C6 glioma cells. (c) Western blot showing expression of wild-type (WT) and mutant Flag-α4 at endogenous levels inα4flMEFs (left). Viable cell growth curves after induction of α4 knockout determined the ability of Flag-α4 mutants to reverse the cell death phenotype caused by α4 knockout (right). For all panels, experiments were repeated three times; representative results are shown. For panelc(right), experiments were performed in triplicate and expressed as mean±s.e.m. Figure 6: The α4 interfaces with the phosphatase are essential for the role of α4 in cell survival. ( a ) Mutational analysis of α4 residues at the interface with both PP2A internal packing and surface residues. Pull-down assay determined the effect of α4 mutations on interaction between α4 and GST-nPP2Ac. Proteins bound to GS4B resin were visualized on SDS–PAGE by coomassie blue staining. ( b ) Co-IP showed defects of recombinant Flag-α4 mutants in binding to cellular PP2Ac in C6 glioma cells. ( c ) Western blot showing expression of wild-type (WT) and mutant Flag-α4 at endogenous levels in α4 fl MEFs (left). Viable cell growth curves after induction of α4 knockout determined the ability of Flag-α4 mutants to reverse the cell death phenotype caused by α4 knockout (right). For all panels, experiments were repeated three times; representative results are shown. For panel c (right), experiments were performed in triplicate and expressed as mean±s.e.m. Full size image We next determined whether the α4 interface mutations affected the function of α4 in cell survival. Wild-type and mutant Flag-tagged α4 were expressed at levels comparable to endogenous α4 in α4 fl MEF cells that stably express a Cre-ER (oestrogen receptor) fusion protein ( Fig. 6c , left panel). Deletion of endogenous α4 was induced by tamoxifen as previously described [23] . As shown by viable cell growth assays ( Fig. 6c , right panel), the cell death phenotype caused by α4 knockout (α4-KO) was reversed by the expression of wild-type Flag-α4, but not by vector control. In contrast, Flag-α4-bearing mutations at either PP2Ac interface, R155E or E214R, could not rescue cell death caused by α4-KO ( Fig. 6c ). These data show that the α4 interface with nPP2Ac is required for α4’s function in cell survival and imply a critical role of phosphatase regulation by α4. Interaction with α4 is essential for PP2Ac stability The previous study showed that knockout of α4 led to a complete loss of total cellular PP2A and PP2A-like phosphatases [23] . To test whether the stability of cellular PP2Ac relies on its interaction with α4, we examined the turnover rate of V5-tagged PP2Ac (V5-C)-bearing mutations that disrupt interaction with α4. The level of V5-C was monitored at different times after addition of cycloheximide to inhibit de novo protein synthesis. Because a large area of the nPP2Ac–α4 interface involves PP2Ac internal packing ( Fig. 4b ), PP2Ac mutations were carefully chosen not to perturb internal packing and were limited to surface residues at the interface with α4. Recombinant wild-type V5-C interacted readily with α4 and exhibited a half-life of about 13 h ( Fig. 7a–c ). V5-C-bearing mutation of PP2Ac surface residues at the interface with α4, Y130D/D131R, failed to interact with α4 ( Fig. 7a ) and exhibited a higher turnover rate ( Fig. 7b ) and a minimum of sixfold reduction in the half-life ( Fig. 7c ). V5-C-bearing mutations outside the interface with α4, K29E, barely affected α4 binding or the cellular stability of PP2Ac ( Fig. 7a–c ). These data indicate that α4 interaction is required for the stability of cellular PP2Ac. 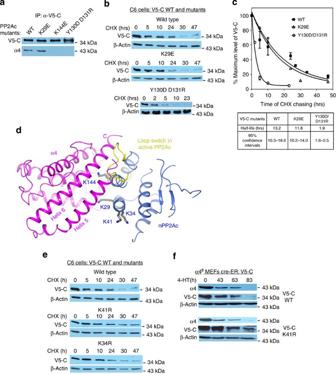Figure 7: The PP2A–α4 interface is essential for the stability of total cellular PP2A. (a) Co-IP determined the interaction between wild-type and mutant V5-C and α4 in C6 glioma cells. (b) Cycloheximide (CHX) chasing and western blot using an antibody that specifically detects V5-tag showed that the turnover rate of V5-C is accelerated by mutations (Y130D/D131R) that disrupt α4 interaction. K29E, a mutation located outside the interface, exhibited no effect. For panelsaandb, experiments were repeated three times; representative results are shown. (c) Exponential decay simulation of the results of CHX chasing described inbdetermined the half-life of wild-type and mutant V5-C. The results shown are the average of three experiments and expressed as mean±s.e.m. (d) Structure of the nPP2Ac–α4 complex highlights PP2A lysine residues (grey) at or near the interface to α4. The loop switch in active PP2Ac is shown (yellow). α4 and nPP2Ac are shown in ribbon and coloured magenta and blue, respectively. (e) CHX chasing showed that the turnover rate of V5-C is reduced by mutation K41R near the interface to α4, but not by K34R. (f) K41R mutation attenuated the loss of V5-C upon α4 knockout. Figure 7: The PP2A–α4 interface is essential for the stability of total cellular PP2A. ( a ) Co-IP determined the interaction between wild-type and mutant V5-C and α4 in C6 glioma cells. ( b ) Cycloheximide (CHX) chasing and western blot using an antibody that specifically detects V5-tag showed that the turnover rate of V5-C is accelerated by mutations (Y130D/D131R) that disrupt α4 interaction. K29E, a mutation located outside the interface, exhibited no effect. For panels a and b , experiments were repeated three times; representative results are shown. ( c ) Exponential decay simulation of the results of CHX chasing described in b determined the half-life of wild-type and mutant V5-C. The results shown are the average of three experiments and expressed as mean±s.e.m. ( d ) Structure of the nPP2Ac–α4 complex highlights PP2A lysine residues (grey) at or near the interface to α4. The loop switch in active PP2Ac is shown (yellow). α4 and nPP2Ac are shown in ribbon and coloured magenta and blue, respectively. ( e ) CHX chasing showed that the turnover rate of V5-C is reduced by mutation K41R near the interface to α4, but not by K34R. ( f ) K41R mutation attenuated the loss of V5-C upon α4 knockout. Full size image α4 was also shown to stabilize PP2Ac and protect it from poly-ubiquitination and degradation [13] , [18] . The structure of the nPP2Ac–α4 complex shows that several lysine residues of PP2Ac are located at or near the interface to α4 ( Fig. 7d ). Among these residues, Lys41 was detected as a ubiquitination site in a global ubiquitination analysis [24] . By cycloheximide-chasing procedure, we showed that V5-C K41R exhibited an extended half-life in C6 cells compared with wild-type V5-C, whereas mutation to another lysine residue, K34R, had no effect on the turnover rate of V5-C ( Fig. 7e ). Upon α4 knockout in α4 fl MEFs, the K41R mutation attenuated the gradual loss of the V5-C caused by α4 knockout ( Fig. 7f ). This result corroborated the notion that K41 is a PP2Ac ubiquitination site and α4 has a role in blocking PP2Ac poly-ubiquitination at this site. Although α4 is critical for the function of all eukaryotic cells and has been intensely investigated for almost two decades, the mechanism of α4 in PP2A regulation and in cellular function has remained enigmatic. In this study, we have shown that the PP2Ac–α4 interaction relies on partial unfolding near the phosphatase active site, and determined the crystal structure of α4 bound to nPP2Ac, a partial PP2Ac encompassing the N-terminal half of PP2Ac. The structure predicts that two structural elements near the phosphatase active site in active PP2Ac, loop switch and helix switch, hinder α4 binding. Displacement of these two structural elements is essential for α4 binding, and associated with two major consequences: distortion of the active site conformation, and allosteric changes that alter the scaffold subunit binding sites at the opposite surface. These structural changes underlie important molecular basis for PP2A latency and exclusive binding of α4 and PP2A scaffold subunit. It is important to note that α4 binding to the partially folded PP2Ac is counterintuitive. All crystal structures of the PPP family serine/threonine phosphatases, including recent structures of PP2A complexes, give similar conformation of the catalytic subunits. The dynamic nature of PP2A active site was suggested in a recent study showing that recombinant PP2Ac could not be fully methylated due to a direct binding of PP2A methyltransferase (LCMT-1) to the active site unless the active site conformation is primed by PP2A phosphatase activator (PTPA) [19] . Insights from the structure of the nPP2Ac–α4 complex are limited by the fact that some of the conformational changes are derived from missing of the C-terminal half of PP2Ac. Nonetheless, the fact that the loop switch is missing and the helix switch is relaxed in the α4-bound nPP2Ac suggests that nPP2Ac resembles partially folded, full-length PP2Ac in α4 binding. To further demonstrate the dynamic nature of PP2Ac in α4 binding, we provided five lines of supporting evidence besides the structural insights derived from the nPP2Ac–α4 complex ( Fig. 4 ): 1) α4 could not bind directly to active PP2Ac; 2) α4 binding blocks aggregation of the inactivated PP2Ac ( Fig. 1a ), presumably by shielding the exposed PP2Ac internal packing; 3) H–D exchange data showed that the PP2A active site loops directly linked to or adjacent to the helix switch are intrinsically dynamic and that the peptide buried by the loop switch and other inner structure in active PP2Ac become more dynamic in the α4-bound PP2Ac ( Fig. 3 ); 4) allosteric relay through central β-sheets ( Fig. 5 ) explains mutually exclusive binding of α4 and the scaffold subunit; 5) α4 contacts with both PP2Ac internal packing and surface residues are essential for α4 interaction with the full-length PP2Ac in cells and the role of α4 in cell survival ( Fig. 6 ). Structural observations suggest that displacement of PP2Ac internal packing for α4 binding is an energetically plausible process. Dynamics of the active site loops and helix switch ( Fig. 3a ) and the increased protein dynamics in the absence of catalytic metal ions would reduce energy barrier of conformational changes required for α4 binding. The energy cost of conformational changes is also compensated by the PP2Ac–α4 interaction that mimics PP2Ac internal packing ( Fig. 4b ). Furthermore, the α4 interface with PP2Ac internal packing is buttressed by contacts with PP2Ac surface residues ( Fig. 4c ). Our studies suggest that binding of α4 with PP2A internal packing near the phosphatase active site underlies elegant mechanisms for stable PP2A latency. α4 binding stabilizes PP2Ac in an inactive conformation, which would suppress the uncontrolled phosphatase activity before formation of substrate-specific phosphatase activity. In addition, α4 binding prevents aggregation of the latent PP2Ac ( Fig. 1b ), and sterically hinders a PP2A ubiquitination site at Lys41 ( Fig. 7 ). These results illuminated dual mechanism of α4 in stabilizing cellular PP2Ac [13] , [18] , and provided the structural basis of α4 in PP2A latency [13] . Stable PP2A latency likely contributes to the role of α4 in cell survival by preventing the cell-detrimental uncontrolled phosphatase activity via stabilizing the free PP2Ac in an inactive form. Stable PP2A latency is crucial for biogenesis of PP2A holoenzymes, which also contributes to cell survival. Loss of PP2A holoenzymes was previously shown to cause cell death [25] , [26] , [27] . The unique mode of α4 binding also suggests an elegant mechanism for mutually exclusive binding of α4 and the scaffold subunit [4] , [5] . These two proteins had been proposed to have overlapping binding site [5] . We showed that the α4-binding site on PP2Ac is opposite from the scaffold subunit-binding site ( Fig. 5a ). This led to a novel model of an extended allosteric relay via the helix switch, the active site loops, the central β-sheet, and the scaffold subunit-binding site linked to the opposite end of the β-sheet ( Fig. 5a ). As a result of this allosteric relay, the binding preferences of PP2Ac are robustly altered, resulting in efficient conversion of PP2A core enzyme and holoenzyme into the PP2Ac–α4 complex upon perturbation of the active site ( Fig. 5b ). The conformational switch of PP2Ac in altering the binding preferences provides an important molecular basis for the recent observation on dissociation of PP2A holoenzymes and recycling of PP2Ac in response to DNA damage response [13] . Recycling of PP2Ac from holoenzymes might be crucial for surveillance of PP2A holoenzymes and regulation of holoenzyme redistribution during cellular signalling. PP2A holoenzyme assembly is believed to be regulated by methylation at a conserved carboxylterminal peptide motif of PP2Ac [28] , [29] , [30] , [31] , [32] . The role of α4 in holoenzyme surveillance is reflected by the fact that defect in PP2A methylation led to increased association between PP2Ac and α4 ( [16] ), presumably due to reduced holoenzyme stability. Protein preparation All constructs and point mutations were generated using a standard PCR-based cloning strategy. The nPP2Ac (1–153), α4 (3–233) and TAP42 (1–234), and their internal deletion constructs and missense mutants were cloned in pQlink vector (Addgene) harbouring a GST- or His 8 -tag and a TEV-cleavage site between the tag and the recombinant protein. The proteins were overexpressed at 23 °C in E. coli strain DH5α. The soluble fraction of the E. coli cell lysate was purified over GS4B resin (GE Healthcare) or Ni-NTA resin (Qiagen), and further fractionated by anion exchange chromatography (Source 15Q, GE Healthcare) and gel filtration chromatography (Superdex 200, GE Healthcare), with or without removal of the affinity tag. Expression and assembly of PP2A core enzyme and holoenzyme follow procedures as previously described [19] , [22] . The nPP2Ac–α4 complex was assembled over GS4B resin with immobilized GST-tagged nPP2Ac bound to α4, followed by cleavage of the GST-tag. The complex was further fractionated by anion exchange and gel filtration chromatography to remove the excess amount of nPP2Ac. Crystallization and data collection Crystals of the nPP2Ac–α4 complex were grown at 20 °C by the sitting-drop vapor-diffusion method by mixing ~8 mg ml −1 of the protein complex with an equal volume of reservoir solution containing 12–15% PEG3350 (v/v), 0.3 M Na/K tartrate. Initial crystals appeared after 1 week and grew poorly. The crystal was improved by seeding and by addition of 10 mM praseodymium acetate (additive), and grew to full within 2 weeks. Crystals were equilibrated in a cryoprotectant buffer containing reservoir buffer with 20% glycerol (v/v), and flash frozen in a cold nitrogen stream at −170 °C. The data sets with anomalous signal of selenium-labelled complex were collected at APS LS-CAT and processed using HKL2000 ( [33] ). Structure determination The structure was determined by SAD (single-wavelength anomalous dispersion) phasing using CRANK [34] in CCP4 [35] . Eight of nine selenium atoms were located by program AFRO/CRUNCH2 [36] and refined using BP3 [37] . Following phase improvement and density modification, a large fraction of α4 and PP2A helix motif was automatically built using Buccaneer [38] . Model errors were corrected manually based on the electron density map followed by manual building of the rest of the model. The structure was built using Coot [39] and refined using REFMAC restraints with TLS [40] . Two TLS groups were used, nPP2Ac and the PP2Ac-binding domain of α4 (3–233). The structure was refined to 2.8 Å, and the free and working R -factors are 22.2% and 17.9%, respectively. GST-mediated pull-down assay To examine the interaction between α4 and PP2Ac or conversion of PP2A core enzyme and holoenzyme to the α4 complex, 10 μg of GST-α4 was mixed with a near stoichiometric amount of free PP2Ac, core enzyme or B′γ1 holoenzyme. The mixture was incubated at 37 °C in the presence or absence of 2 mM PPi or 50 μM Mn ++ for the indicated period of time in 200 μl of assay buffer containing 25 mM Tris (pH 8.0), 150 mM NaCl, 2 mM dithiothreitol and 1 mg ml −1 BSA to block non-specific binding. The sample was then bound to 10 μl of GS4B resin via GST-tag. After three washes with the assay buffer, the proteins bound to the resin were examined by SDS–PAGE, and visualized by Coomassie blue staining. Alternatively, 10 μg of GST-nPP2Ac was bound to 10 μl of GS4B resin followed by three washes to remove unbound protein. Ten micrograms of wild-type or mutant α4 was bound to the resin as described above. All experiments were repeated three times; representative results are shown. Phosphatase assays PP2A phosphatase activity was measured using a phospho-Thr peptide. Briefly, 2 μl of 1 mM phosphopeptide substrate (K-R-pT-I-R-R) was added to 20 μl of PP2A sample (20–100 nM). The reaction was performed at 30 °C for 15 min and stopped by addition of 50 μl of malachite green solution. The absorbance at 620 nm was measured after 10 min incubation at room temperature. All experiments were performed in triplicate and repeated three times. Mean±SEM were calculated. Isothermal titration calorimetry To obtain a direct binding affinity between α4 and nPP2Ac, 400 μM of α4 was titrated with 20 μM of nPP2Ac using a VP-ITC microcalorimeter (MicroCal). All proteins were prepared in a buffer containing 20 mM HEPES (pH 8.0) and 100 mM NaCl. The data were fitted by Origin 7.0. Determination of metal ion content of PP2Ac The mixtures of active PP2Ac (0.3 mg) and α4 (0.3 mg) were incubated with 50 μM Mn ++ or 3 mM PPi at 37 °C for 10 min, followed by removal of PPi and unbound Mn ++ ions by gel filtration chromatography. Metal contents of both PP2A samples were then determined by ICP-MS. Re-activation of the inactive PP2Ac–α4 complex induced by PPi was performed by co-incubation with 50 μM Mn ++ ions, followed by determination of the phosphatase activity and metal content as described above. H–D exchange mass spectrometry H–D exchange was performed following a similar procedure as described [41] . Briefly, 40 μl PP2Ac (2 mg ml −1 ) bound to Mn ++ or with α4 in D 2 O containing 10 mM HEPES, pD 8.0, 50 mM NaCl, and 1 mM dithiothreitol was incubated at 37 °C for 10 min to allow deuterium intake into residues with exposed backbone amide. PP2Ac bound with α4 was induced by co-incubation with 1 mM PPi. The samples were incubated for another 30 min at room temperature, followed by addition of 5 μl 0.5 M sodium citrate (pH 2.4) on ice to quench H–D exchange and pepsin digestion for 5 min. Pepsin cleavage was stopped by addition of 1 μl of pepstatin A (2 mM) and immediate freezing in liquid nitrogen. PP2Ac without H–D exchange was used as control. Control sample was characterized both by liquid chromatography-MS to obtain the control spectra and by tandem MS (TOF/TOF) to confirm the peptide sequences of pepsin-cleaved PP2A fragments. PP2A samples that underwent H–D exchange were analysed by liquid chromatography-MS, and spectra were compared with control to determine the level of backbone amide deuterium intake into PP2Ac. The spectra of PP2Ac fragments were analysed using software Mass Hunter (Agilent Technologies), and the level of deuterium intake was calculated using Excel-based software HXExpress downloaded from http://www.hxms.com/HXExpress( [42] ). Ratio of deuterium intake by PP2Ac bound to α4 versus PP2Ac bound to Mn ++ for each peptide was used to evaluate increased dynamics in α4-bound PP2Ac. Mammalian cell culture and western blot The Flag-tagged human α4 (Flag-α4), V5-tagged human PP2A catalytic subunit α isoform (V5-C) and their missense mutants were cloned into murine leukaemia retroviral vectors harbouring a CMV promoter for overexpression, or a PGK promoter for expression at endogenous levels. 293T, C6 glioma cells and MEFs harbouring conditional α4 knockout α 4 fl and stable Cre-ER [23] were cultured in Dulbecco’s modified Eagle’s medium supplemented with 10% fetal bovine serum, 100 units per ml of penicillin and 100 μg ml −1 of streptomycin. Retroviruses harbouring the recombinant gene were packaged in 293T cells, and the same titre of retroviruses was used to infect cells with 50–80% confluence for expression of Flag-α4, V5-C and their mutants. Knockout of α4 was induced by addition of 200 nM 4-hydroxytamoxifen (4-HT) (Sigma) to α 4 fl MEFs Cre-ER [23] . The infection efficiency of retroviruses was monitored by the fluorescence signals of RFP or GFP included in retroviral vectors. The expression level of recombinant and endogenous proteins was monitored by western blot using antibodies that specifically recognize Flag-tag (Sigma, M2), V5-tag (Millipore), α4 (Millipore, 5F6) or PP2A Cα subunit (Millipore, 1D6). For loading control, cell extracts with equal amounts of protein (10–50 μg) were detected by western blot using an antibody that specifically recognizes actin (Millipore, C4). Co-immunoprecipitation (co-IP) The interaction between wild-type or mutant Flag-α4 and PP2Ac was determined by co-IP using anti-FLAG M2 affinity gel (Sigma, A2220) to immunoprecipitate PP2Ac. The level of Flag-α4 and the associated PP2Ac were determined by western blot as described above. Similarly, the interaction between V5-C and α4 was determined by co-IP using anti-V5 antibody (Millipore) and the associated PP2Ac subunit was detected by western blot as described above. All experiments were repeated three times; representative results are shown. Cell viability assay Cell death caused by knockout of α4 was determined using viable cell assays. Briefly, the same number of α4fl MEFs Cre-ER cells that stably express Flag-α4 or its mutants were placed into 96-well plates (~1,000 cells per well). Proliferation of viable cells was determined using the CellTiter-Glo luminescent cell viability assay (Promega) 24 h after induction of α4-KO at the indicated time. The experiments were performed in triplicate and repeated at least three times. Mean±s.e.m. were calculated. Cycloheximide-chasing experiment C6 cells that stably express wild-type or mutant V5-C were mixed with 100 μg ml −1 cycloheximide (Sigma) and passed into six-well plates with about 5 × 10 5 cells per well. The cells were collected at the indicated time and the level of V5-C was monitored by western blot using the antibody that specifically recognizes the V5-tag. Actin was detected by western blot as a loading control. All experiments were repeated three times. The data were fitted in GraphPad Prism to calculate the half-life of V5-C. Mean±s.e.m. were calculated. Accession codes: the atomic coordinates of the nPP2Ac–α4 complex have been deposited in the Protein Data Bank under accession code 4IYP . How to cite this article: Jiang, L. et al . Structural basis of protein phosphatase 2A stable latency. Nat. Commun. 4:1699 doi: 10.1038/ncomms2663 (2013).